Action of the Hsp70 chaperone system observed with single proteins In Escherichia coli , the binding of non-native protein substrates to the Hsp70 chaperone DnaK is mediated by the co-chaperone DnaJ. DnaJ accelerates ATP hydrolysis on DnaK, by closing the peptide-binding cleft of DnaK. GrpE catalysed nucleotide exchange and ATP re-binding then lead to substrate release from DnaK, allowing folding. Here we refold immunoglobulin 27 (I27) to better understand how DnaJ-DnaK-GrpE chaperones cooperate. When DnaJ is present, I27 is less likely to misfold and more likely to fold, whereas the unfolded state remains unaffected. Thus, the ‘holdase’ DnaJ shows foldase behaviour. Misfolding of I27 is fully abrogated when DnaJ cooperates with DnaK, which stabilizes the unfolded state and increases the probability of folding. Addition of GrpE shifts the unfolded fraction of I27 to pre-chaperone levels. These insights reveal synergistic mechanisms within the evolutionary highly conserved Hsp70 system that prevent substrates from misfolding and promote their productive transition to the native state. Most newly synthesized proteins must fold into well-defined three-dimensional conformations in order to become functionally active. Non-native protein chains are often prone to aggregation because of the exposure of hydrophobic sequences that are buried in the folded structure. Aggregation is promoted by the high concentration of macromolecules in the cellular environment [1] , [2] . Protein folding in vivo often requires the assistance of molecular chaperones that recognize and shield exposed hydrophobic stretches in non-native proteins and thereby prevent misfolding and aggregation [2] . The Hsp70 chaperone system has an important role in binding nascent polypeptide chains on ribosomes, stabilizing them in a folding-competent, non-aggregated state until sufficient structural information for folding is available [2] . The E. coli Hsp70 chaperone homologue, DnaK, is the best studied representative of this chaperone class [3] , [4] , [5] . DnaK assists protein folding through cycles of ATP-dependent substrate binding and release [3] , [5] . Hydrolysis of ATP drives conformational changes in a peptide-binding cleft located in the C-terminal domain of DnaK that lead to the entrapment of peptide substrates [5] . Following dissociation of the newly formed ADP, re-binding of ATP opens the binding cleft and allows substrate release [6] . Efficient hydrolysis of DnaK-bound ATP and substrate capture depends upon the functional cooperation of the co-chaperone DnaJ [7] , [8] . Furthermore, cycling of substrate between bound and free states requires the nucleotide exchange factor GrpE [5] . DnaJ, a dimer of ≈40 kDa subunits, possesses autonomous chaperone activity in binding and stabilizing unfolded proteins [3] , [5] , [9] , [10] , [11] , [12] . DnaJ is able to bind substrates with fewer steric constraints than DnaK and serves as a substrate selector for DnaK [13] , [14] . As DnaJ has no ATPase activity, it functions as a ‘holdase’ and does not actively promote refolding. This is supported by experimental observations of a pronounced inhibitory effect of DnaJ binding to unfolded luciferase [15] and rhodanese [9] , while preventing these proteins from aggregating [5] , [9] , [15] . Refolding or transfer to downstream chaperones, such as the cylindrical chaperonin GroEL [16] , then occurs in the presence of DnaK, ATP and GrpE [4] , [5] . The Hsp70 system in E. coli has been studied using either protein substrates with relatively complex structures, such as bovine rhodanese [3] , [9] and luciferase [4] , [9] , [15] , or with proteins lacking stable structure, such as αS1-casein and carboxy-methylated-α-lactalbumin [3] . However, mechanistic details may be obscured either by the inherent complexity of substrates or by the lack thereof. Here we have used the immunoglobulin 27 (I27) domain of the human striated muscle protein titin as a model substrate to obtain insight into the function of the Hsp70 chaperone system. I27 is an 89 amino-acid single-domain protein with a molecular weight of ≈10 kDa. As a member of the immunoglobulin superfamily, it has the typical immunoglobulin fold, which consists of a ‘sandwich’ of two β-sheets with a Greek key topology each composed of seven to nine anti-parallel β-strands [17] . Mechanical unfolding of multiple immunoglobulin titin domains using single-molecule force spectroscopy (SMFS) records a well-defined ‘saw-tooth’ pattern, allowing properly folded single immunoglobulin domains to be identified [18] , [19] . Force and fluorescence spectroscopy experiments on engineered I27 homomeric repeats have shown that the I27 domain folds at a rate of ≈1.2 s −1 (ref. 20 ). Recent studies using Förster resonance energy transfer [21] and light scattering [22] have characterized misfolding and aggregation of I27 in a similar context, allowing both folding and misfolding pathways to be explored simultaneously. I27 has been previously used to study the chaperone trigger factor [23] , indicating its potential utility in the study of other chaperone systems. Here we employed atomic force microscopy (AFM)-based SMFS to study the action of the E. coli Hsp70 system in assisting the folding of an I27 octomer (8xI27) under physiologically relevant solvent conditions. The central finding of our experiments is that the holdase DnaJ can show foldase behaviour. We characterized 8xI27 as a fast-folding high-aggregation system and observed that unfolded conformations of I27 are less likely to misfold and aggregate in the presence of DnaJ. Interestingly, this is not achieved by shifting the equilibrium towards the unfolded state. Instead, DnaJ appears to constrain the conformational space that is explored during folding, thus reducing the probability of misfolding and increasing the probability of correct folding. In contrast, when DnaJ and DnaK are combined in the presence of ATP, the unfolded state is stabilized at the expense of the misfolded state. This stabilized unfolded state depletes the substrate misfolded states and further populates the folded state. Adding GrpE to DnaJ and DnaK reduces the population of unfolded I27 conformations to pre-chaperone levels and marginally increases the folded and misfolded populations, an observation consistent with accelerating protein release from DnaK. 8xI27 is a substrate suitable for studying the Hsp70 system Our refolding experiments consist of an SMFS experiment with three distinct phases. First, a folded 8xI27 tethered to a gold support ( Fig. 1a ) is extended at constant speed (1,200 nm s −1 ) until unfolded ( Fig. 1b ). The unfolded 8xI27 polypeptide is then approached back to the support for a defined refolding time ( t r ). During this period, I27 domains can undergo refolding. Finally, 8xI27 is unfolded once again at constant speed (1,200 nm s −1 ). Comparison of force data obtained for the two unfolding phases provides information about the type of folding reaction, its kinetics and its yield. Properly folded I27 domains can be identified in force-distance curves because of their well-defined unfolding force peaks ( Fig. 1b ). Force peaks were fitted using the worm-like chain model to estimate unfolding forces and contour lengths associated with I27 conformers ( Fig. 1c ). Based on force-distance curves obtained from unfolding 8xI27, folded conformers are defined as I27 domains where the contour lengths separating individual unfolding force peaks are between 25 and 31 nm and unfolding forces ( F ) are between 50 and 300 pN ( Supplementary Fig. 1 ). The absence of force features corresponding to a particular I27 domain indicates that the domain did not refold and therefore remains in the unfolded conformation ( Fig. 1b,c ). Analysis of force-distance curves from refolded 8xI27 suggests that some I27 domains adopt conformations that are neither folded nor unfolded ( Fig. 1c ). The presence of force features that do not meet the criteria for properly folded I27 domains are considered to denote domain misfolding ( Fig. 1c ). 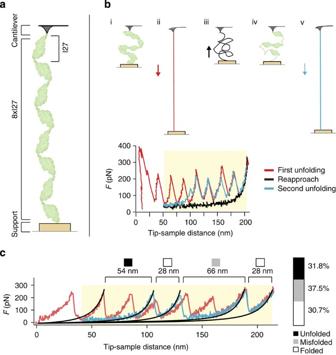Figure 1: Mechanical characterization of I27 conformers. (a) Illustration of 8xI27 (green domains) tethered by the C-terminus to a gold support and N-terminally attached to the tip of the AFM cantilever. (b) Example of force-distance curves recorded upon initial unfolding and after refolding a single 8xI27, accompanied by explanatory illustrations (i–v). 8xI27 (i) is unfolded (ii) when retracting the support (red arrow), rendering the red force-distance curve. Each force peak of the force-distance curve corresponds to the unfolding of a single I27 domain. Thereafter, the tension applied to unfold I27 domains is reduced by re-approaching tip and support indicated by the black arrow (iii), resulting in the black force-distance curve. The collapsed unfolded 8xI27 (iii) is kept relaxed for a given refolding time (1–8 s). During this period some I27 domains may refold (iv). To characterize the adopted conformations, the same protein is once again unfolded (v). The resulting turquoise force-distance curve shows the number of domains refolded (in this example four I27 domains). To avoid unspecific interactions between tip and support, the tip is kept separated from the support by ≈20 nm (close to the contour length of one unfolded I27 domain). The portion of 8xI27 allowed to refold is highlighted by the light yellow background of the force-distance curves. (c) Identifying different I27 conformers in force-distance curves recorded upon initial unfolding (red) and unfolding refolded 8xI27 (turquoise). Force peaks were fitted using the worm-like chain (WLC) model to reveal contour lengths and unfolding forces (black fits). The contour length difference between force peaks is used to characterize I27 conformers. Folded conformers (white squares) are found to have contour lengths separating individual force peaks between 25 and 31 nm and unfolding forces (F) between 50 and 300 pN. Force features that do not meet criteria for properly folded I27 domains originate from misfolded I27 conformers (grey squares). The absence of force features preceding the first force peak reflect I27 domains that did not refold and therefore indicate unfolded conformations (black squares). The bar represents the percentage of I27 conformers detected by the refolding force-distance curve (turquoise). Figure 1: Mechanical characterization of I27 conformers. ( a ) Illustration of 8xI27 (green domains) tethered by the C-terminus to a gold support and N-terminally attached to the tip of the AFM cantilever. ( b ) Example of force-distance curves recorded upon initial unfolding and after refolding a single 8xI27, accompanied by explanatory illustrations (i–v). 8xI27 (i) is unfolded (ii) when retracting the support (red arrow), rendering the red force-distance curve. Each force peak of the force-distance curve corresponds to the unfolding of a single I27 domain. Thereafter, the tension applied to unfold I27 domains is reduced by re-approaching tip and support indicated by the black arrow (iii), resulting in the black force-distance curve. The collapsed unfolded 8xI27 (iii) is kept relaxed for a given refolding time (1–8 s). During this period some I27 domains may refold (iv). To characterize the adopted conformations, the same protein is once again unfolded (v). The resulting turquoise force-distance curve shows the number of domains refolded (in this example four I27 domains). To avoid unspecific interactions between tip and support, the tip is kept separated from the support by ≈20 nm (close to the contour length of one unfolded I27 domain). The portion of 8xI27 allowed to refold is highlighted by the light yellow background of the force-distance curves. ( c ) Identifying different I27 conformers in force-distance curves recorded upon initial unfolding (red) and unfolding refolded 8xI27 (turquoise). Force peaks were fitted using the worm-like chain (WLC) model to reveal contour lengths and unfolding forces (black fits). The contour length difference between force peaks is used to characterize I27 conformers. Folded conformers (white squares) are found to have contour lengths separating individual force peaks between 25 and 31 nm and unfolding forces ( F ) between 50 and 300 pN. Force features that do not meet criteria for properly folded I27 domains originate from misfolded I27 conformers (grey squares). The absence of force features preceding the first force peak reflect I27 domains that did not refold and therefore indicate unfolded conformations (black squares). The bar represents the percentage of I27 conformers detected by the refolding force-distance curve (turquoise). Full size image To probe the refolding of I27, we unfolded and refolded 8xI27 constructs many times ( n =60) in the absence of chaperones ( Fig. 2a ). The number of I27 domains in each conformation were counted as described above and statistically analysed ( Supplementary Table 1 ). The refolding experiments show that misfolding is the dominant process, and an average of ≈54% of all I27 domains ( n =405) are misfolded at steady state ( Fig. 2a and Supplementary Fig. 2 ). The steady state of all three I27 conformations is approached at a refolding time of 5 s ( Supplementary Fig. 2 ). At this steady state, ≈25% of all I27 domains remained in the unfolded state ( Fig. 2a ), which is consistent with the kinetic delay observed in folding of an unfolded protein subjected to mechanical strain [20] . Such strain was applied in our experiments to minimize unspecific interactions of the unfolded 8xI27 construct with the surfaces of the AFM tip or/and the gold support. More specifically, as we kept the unfolded 8xI27 construct separated by ≈20 nm from the gold support ( Fig. 1 ), the applied tension is expected to shift the fraction of I27 domains that remain unfolded to ≈20% at refolding times of 5 s (ref. 20 ). 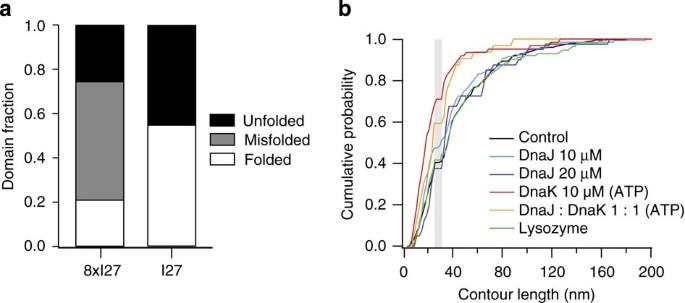Figure 2: Nature of misfolded conformers. (a) Fraction of I27 domains attaining unfolded, misfolded and folded conformations upon refolding 8xI27 (n=405) and single I27 (n=25). The refolding data of single I27 domains is the result of experiments performed at different refolding times. The refolding data of 8xI27 have been recorded at steady-state refolding conditions (refolding time 5 s,Supplementary Fig. 2). (b) Cumulative probability distribution of contour lengths of misfolded I27 conformers from steady-state experiments. The binning used was 2 nm. The black line represents control data (n=217), light blue line represents data obtained in the presence of 10 μM DnaJ (n=193), purple line represents data obtained in the presence of 20 μM DnaJ (n=63), red line represents data obtained in the presence of 10 μM DnaK and ATP (n=64), yellow line represents data obtained in the presence of 10 μM DnaK, 10 μM DnaJ and ATP (n=31), green line represents data obtained in the presence of 20 μM lysozyme (n=197). The grey shaded area represents the contour length (28±3 nm,Supplementary Fig. 1c) of one unfolded I27 domain. Figure 2: Nature of misfolded conformers. ( a ) Fraction of I27 domains attaining unfolded, misfolded and folded conformations upon refolding 8xI27 ( n =405) and single I27 ( n =25). The refolding data of single I27 domains is the result of experiments performed at different refolding times. The refolding data of 8xI27 have been recorded at steady-state refolding conditions (refolding time 5 s, Supplementary Fig. 2 ). ( b ) Cumulative probability distribution of contour lengths of misfolded I27 conformers from steady-state experiments. The binning used was 2 nm. The black line represents control data ( n =217), light blue line represents data obtained in the presence of 10 μM DnaJ ( n =193), purple line represents data obtained in the presence of 20 μM DnaJ ( n =63), red line represents data obtained in the presence of 10 μM DnaK and ATP ( n =64), yellow line represents data obtained in the presence of 10 μM DnaK, 10 μM DnaJ and ATP ( n =31), green line represents data obtained in the presence of 20 μM lysozyme ( n =197). The grey shaded area represents the contour length (28±3 nm, Supplementary Fig. 1c ) of one unfolded I27 domain. Full size image The results obtained from refolding 8xI27 ( Fig. 2a ) differ from previous reports that 8xI27 mainly refolds and rarely misfolds [20] , [24] but are in accord with observations of misfolding and aggregation in other studies [21] , [22] . All four studies used PBS as a buffer and I27 substrates but differed on the techniques used to study folding. More specifically refs 20 and 24 used SMFS and 8xI27 as a substrate. [21] used Förster resonance energy transfer to study the folding of monomeric I27, 2xI27 and 3xI27 and ref. 22 used light scattering and fluorescence spectroscopy to characterize the folding of monomeric I27, 2xI27, 3xI27 and 8xI27. To investigate how misfolding occurs in the multi-domain fusion protein 8xI27, we subjected single I27 domains to refolding experiments while restricting the refolding length ( z r ) of 8xI27 to ≈40 nm. The result is that single I27 domains do not misfold and thus adopt one of two possible conformations: folded or unfolded ( Fig. 2a ). Furthermore, the contour lengths of misfolded 8xI27 conformers display a broad distribution ( Fig. 2b ). This broad distribution is most likely due to the high number of possible misfolded conformations. About half of the unfolding force peaks show contour lengths greater than that of a single I27 domain, suggesting that these misfolding events occur through aggregation of two or more adjacent unfolded I27 domains. Furthermore, the observed broad contour length distribution for misfolded conformers is in agreement with previous studies on misfolding and aggregation of I27 (refs 21 , 22 ). Our SMFS setup thus provides single-domain resolution and can differentiate between folded, unfolded and misfolded conformers ( Fig. 1c ) and ultimately reveals that 8xI27 is an aggregation-prone system ( Fig. 2a and Supplementary Fig. 2 ). DnaJ suppresses misfolding and promotes folding To determine DnaJ’s effect on 8xI27 folding, the SMFS-based refolding experiments were repeated with the addition of DnaJ to the medium. Physiological DnaJ concentrations recorded in E. coli vary between 10 and 30 μM (ref. 25 ). Thus, we refolded 8xI27 at DnaJ concentrations between 1 and 20 μM in the absence of ATP ( Supplementary Fig. 3 ). A linear increase in the yield of the folded conformation is observed for DnaJ concentrations >5 μM. Surprisingly, this increase in folded I27 is obtained at the expense of the misfolded population, whereas the proportion of unfolded I27 remains unchanged compared with control conditions in the absence of chaperones ( Supplementary Fig. 3 ). For instance, with DnaJ present at a concentration of 10 μM, the mean fraction of folded I27 increases from 0.21±0.03 (mean±standard error, n =405) to 0.35±0.04 ( n =479), whereas the fraction of misfolded I27 reduces from 0.54±0.03 ( n =405) to 0.40±0.04 ( n =479; Fig. 3 ). In summary, these experiments nicely demonstrate that the transition of misfolding I27 conformers to folded conformers linearly increases with the DnaJ concentration. To test whether this effect is specific to DnaJ, we unfolded and refolded I27 in the presence of 20 μM lysozyme thereby approaching the maximum concentration of DnaJ tested. No significant differences were observed between data sets recorded in the absence and presence of lysozyme. 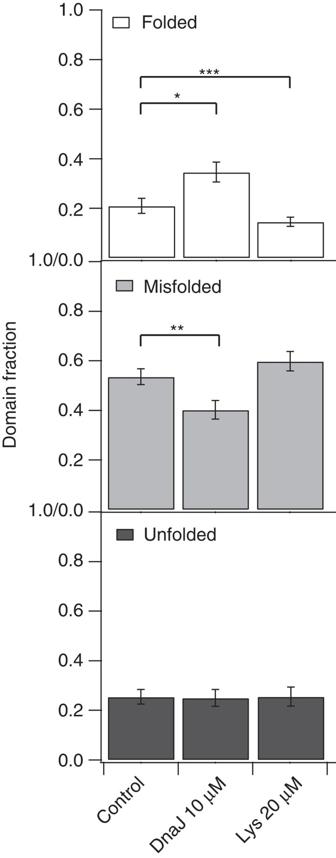Figure 3: DnaJ limits misfolding and assists folding. Average domain fractions (white—folded, grey—misfolded and black—unfolded) obtained in the presence of 10 μM DnaJ were compared at steady state with control experiments using 8xI27 alone (control) or in the presence of 20 μM lysozyme (Lys). The number of domains analysed was 405 for control, 479 for 10 μM DnaJ and 329 for lysozyme. *P≤0.05, **P≤0.01 and ***P≤0.001, withP-values determined using the Mann–WhitneyU-test are given inSupplementary Table 2. Error bars represent the standard error (s.e.). Figure 3: DnaJ limits misfolding and assists folding. Average domain fractions (white—folded, grey—misfolded and black—unfolded) obtained in the presence of 10 μM DnaJ were compared at steady state with control experiments using 8xI27 alone (control) or in the presence of 20 μM lysozyme (Lys). The number of domains analysed was 405 for control, 479 for 10 μM DnaJ and 329 for lysozyme. * P ≤0.05, ** P ≤0.01 and *** P ≤0.001, with P -values determined using the Mann–Whitney U -test are given in Supplementary Table 2 . Error bars represent the standard error (s.e.). Full size image Analysis of the unfolding forces of folded 8xI27 showed that the stability of immunoglobulin was not affected by the presence of chaperones or other cofactors ( Supplementary Fig. 4 ). For all DnaJ concentrations, the contour lengths of misfolded I27 conformers were similarly distributed to those measured in the absence of chaperones ( Fig. 2b ). These results suggest that DnaJ does not affect the type of interactions stabilizing folded and misfolded I27 domains. In summary, the refolding experiments showed that chaperoning by DnaJ promotes protein folding while decreasing the fraction of misfolded I27 domains but the fraction of unfolded domains is unaffected. DnaJ synergizes with DnaK to assist folding One important role ascribed to DnaJ is to function as a substrate selector for DnaK [12] , [14] . Therefore, we also performed refolding experiments on 8xI27 in the presence of DnaK alone, and in the presence of DnaJ and DnaK ( Fig. 4 ). The steady-state profiles of I27 conformers recorded in the presence of DnaK and ATP show significantly reduced populations of the unfolded state and a slight increase of folded and misfolded conformers ( Fig. 4 and Supplementary Table 2 ). The contour length distribution for misfolded conformers reveals that 94% presented an extension less than that of two unfolded I27 domains (<56±6 nm, Fig. 2b ). In previous experiments, it was shown that the binding and unbinding kinetics of DnaK is not related to ATP hydrolysis [6] , [13] , [26] . To test this hypothesis we conducted control experiments refolding 8xI27 in the presence of DnaK with and without ATP ( Supplementary Fig. 5 ). The results of these controls are in excellent agreement with the hypothesis that the activity of DnaK alone is not associated with ATP hydrolysis. However, to study how the combination of DnaJ and DnaK modulates these folding and misfolding processes, 8xI27 was refolded in the presence of both chaperones. The fraction of folded conformers increased from DnaJ/DnaK ratios of 1:0, 1:1 to 1:2 where they reach a maximum of ≈0.7 (70%) at steady state ( Fig. 4 ). Interestingly, as the DnaJ/DnaK ratio was further decreased to 1:100, the fraction of folded conformers again reduced and that of the unfolded conformers increased to nearly 50%. 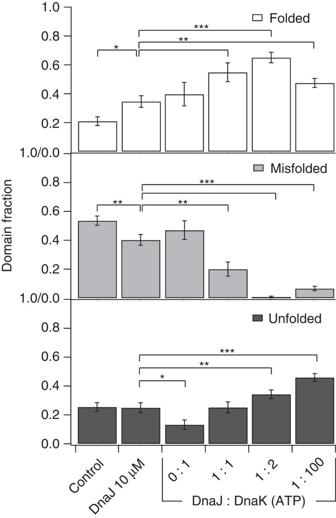Figure 4: Effect of DnaJ on DnaK efficiency in stabilizing unfolded I27 domains and guiding their folding. Individual plots were generated for folded (white bars), misfolded (grey bars) and unfolded (black bars) average fractions recorded at steady-state refolding conditions (tr=5 s). The number of domains analysed was 405 for control, 479 for 10 μM DnaJ, 136 for 10 μM DnaK, 155 for 1:1 DnaJ/DnaK (10 μM DnaJ, 10 μM DnaK), 169 for 1:2 DnaJ/DnaK (5 μM DnaJ, 10 μM DnaK) and 274 for 1:100 DnaJ/DnaK (0.1 μM DnaJ, 10 μM DnaK). Refolding experiments were conducted in the presence of 2 mM ATP except for the control and DnaJ alone. *P≤0.05, **P≤0.01 and ***P≤0.001, withP-values determined using the Mann–WhitneyU-test are given inSupplementary Table 2. Error bars represent the standard error (s.e.). Figure 4: Effect of DnaJ on DnaK efficiency in stabilizing unfolded I27 domains and guiding their folding. Individual plots were generated for folded (white bars), misfolded (grey bars) and unfolded (black bars) average fractions recorded at steady-state refolding conditions ( t r =5 s). The number of domains analysed was 405 for control, 479 for 10 μM DnaJ, 136 for 10 μM DnaK, 155 for 1:1 DnaJ/DnaK (10 μM DnaJ, 10 μM DnaK), 169 for 1:2 DnaJ/DnaK (5 μM DnaJ, 10 μM DnaK) and 274 for 1:100 DnaJ/DnaK (0.1 μM DnaJ, 10 μM DnaK). Refolding experiments were conducted in the presence of 2 mM ATP except for the control and DnaJ alone. * P ≤0.05, ** P ≤0.01 and *** P ≤0.001, with P -values determined using the Mann–Whitney U -test are given in Supplementary Table 2 . Error bars represent the standard error (s.e.). Full size image The efficiency of the DnaJ-DnaK system was optimal at a DnaJ/DnaK ratio of 1:2, preventing misfolding almost entirely (<1%) and significantly increasing the population of the unfolded state to one-third of all I27 domains at steady state. For ratios lower than 1:2, no significant increase in the fraction of misfolded conformers was observed. Closer inspection of contour lengths arising from misfolded conformers at equimolar DnaJ/DnaK ratio reveals a cumulative distribution similar to that obtained for DnaK alone ( Fig. 2b ). This indicates that in the presence of DnaK the contour length of the misfolded conformers is significantly reduced and therefore the propensity of misfolded conformers to aggregate is decreased. No contour length distributions of misfolded conformers were obtained for any other ratios of both chaperones because of the low number of misfolded conformers ( Fig. 4 and Supplementary Table 1 ). Addition of GrpE to experiments in the presence of DnaJ and DnaK tends to lower the fraction of unfolded state to control levels, and marginally increases the fraction of folded and misfolded I27 conformers ( Fig. 5 ). This effect observed for the Hsp70 chaperoning system is consistent with accelerating substrate release from DnaK [5] . 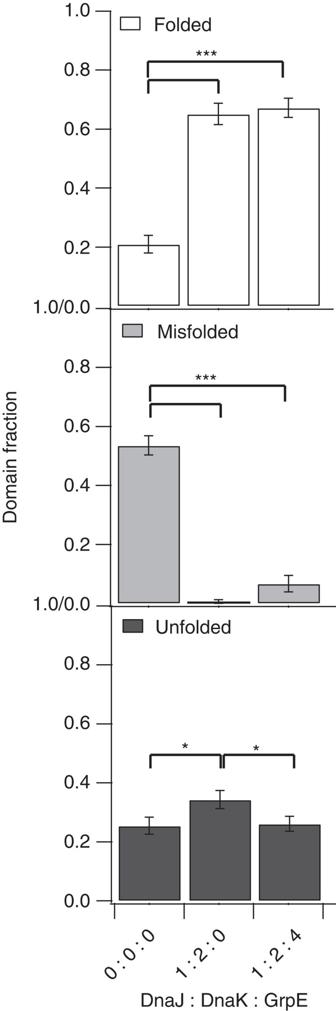Figure 5: GrpE rescues stabilization of unfolded conformers induced by a 1:2 pairwise combination of DnaJ/DnaK. Steady-state (refolding time 5 s) profiles obtained from refolding experiments conducted in the absence of chaperones (control), in the presence of 5 μM DnaJ and 10 μM DnaK, and in the presence of 5 μM DnaJ, 10 μM DnaK and 20 μM GrpE. White bars stand for folded conformations, black bars for unfolded conformations and grey bars for misfolded conformations. Number of I27 domains analysed was 405 for control (0:0:0=DnaJ/DnaK/GrpE), 169 for 5 μM DnaJ and 10 μM DnaK (1:2:0=DnaJ/DnaK/GrpE) and 134 for 5 μM DnaJ, 10 μM DnaK and 20 μM GrpE (1:2:4=DnaJ/DnaK/GrpE). The refolding data were recorded in the presence of ATP. *P≤0.05, **P≤0.01 and ***P≤0.001, withP-values determined using the Mann–WhitneyU-test are given inSupplementary Table 2. Error bars represent the standard error (s.e.). Figure 5: GrpE rescues stabilization of unfolded conformers induced by a 1:2 pairwise combination of DnaJ/DnaK. Steady-state (refolding time 5 s) profiles obtained from refolding experiments conducted in the absence of chaperones (control), in the presence of 5 μM DnaJ and 10 μM DnaK, and in the presence of 5 μM DnaJ, 10 μM DnaK and 20 μM GrpE. White bars stand for folded conformations, black bars for unfolded conformations and grey bars for misfolded conformations. Number of I27 domains analysed was 405 for control (0:0:0=DnaJ/DnaK/GrpE), 169 for 5 μM DnaJ and 10 μM DnaK (1:2:0=DnaJ/DnaK/GrpE) and 134 for 5 μM DnaJ, 10 μM DnaK and 20 μM GrpE (1:2:4=DnaJ/DnaK/GrpE). The refolding data were recorded in the presence of ATP. * P ≤0.05, ** P ≤0.01 and *** P ≤0.001, with P -values determined using the Mann–Whitney U -test are given in Supplementary Table 2 . Error bars represent the standard error (s.e.). Full size image The I27 domain of human titin, expressed as an 8xI27 multi-domain protein, serves as a suitable model for studying the E. coli Hsp70 system by force spectroscopy ( Fig. 1 ). Our results show that 8xI27 is a fast-folding system ( Supplementary Fig. 2 ) that is amenable to single-domain resolution spectroscopy ( Fig. 1 ) and can be modulated by the chaperones being studied ( Figs 2 and 4 ). We demonstrate that 8xI27 is prone to intramolecular aggregation ( Fig. 2a and Supplementary Fig. 2 ). Refolding kinetics show that misfolding is the predominant outcome, amounting to ≈54% of all I27 domains at steady state ( Supplementary Fig. 2 ). Therefore, 8xI27 is a system where both folding and misfolding pathways can be simultaneously explored. The effect of chaperones on the steady-state folding equilibrium of I27 domains was investigated. Previously, DnaJ was categorized as a holdase because of its inhibitory effect on refolding while serving as a deterrent to misfolding and aggregation [4] , [9] , [15] . Surprisingly, at the single-molecule level, DnaJ increases successful folding at the expense of misfolding, whereas the fraction of unfolded conformers remains identical to that found in the absence of chaperones ( Fig. 3 and Supplementary Fig. 3 ). This indicates that DnaJ supports the folding process. Considering that DnaJ binds to proteins in the unfolded conformation [3] , [5] , [9] , the direct conversion of misfolded into folded conformers must be an unlikely event within biologically relevant timescales. Furthermore, the contour length distribution of misfolded conformers remains similar to controls, precluding a mechanism that might process misfolded to folded conformers ( Fig. 2b ). It is thus likely that DnaJ constrains the conformational space of unfolded I27 to prevent unfolded domains from misfolding and aggregating. However, although DnaJ stabilizes the unfolded state, it allows unfolded conformers to preferentially convert into folded conformers. Our observations are consistent with previous findings that DnaJ has a stabilizing effect during multi-domain protein folding [4] , [9] , [15] . As the conformational space surrounding unfolded substrates is constrained by DnaJ, side reactions are impaired and formation of the native tertiary structure is facilitated. Previous publications have shown that DnaK in the presence of ATP has fast unbinding kinetics and even faster binding kinetics [27] . This activity is not associated with ATP hydrolysis as the ATPase activity of DnaK is several orders of magnitude slower [6] . Our results show that DnaK upon binding of ATP reduces the fraction of unfolded I27 conformers, thereby increasing the fraction of misfolded and folded conformers ( Fig. 4 ). Although DnaK can hinder interaction between remotely located domains, it cannot prevent misfolding ( Figs 2b and 4 ). Experiments were conducted in the presence of DnaK and DnaJ to investigate their synergistic effects. Because an increase in the concentration of DnaJ may hinder the efficiency of the chaperone pair, different ratios were tested [7] . The general trend is that the smaller the DnaJ/DnaK ratio, the greater is the fraction of unfolded conformers. Based on this result, we can conclude that DnaJ and DnaK together stabilize the unfolded state in the presence of ATP [5] . Optimal refolding, however, was achieved with DnaJ/DnaK ratios of 1:2, as the fraction of folded conformers is maximized while misfolding is almost eradicated, with <1% conformers misfolded at steady state ( Fig. 4 ). If the DnaJ/DnaK ratio is progressively lowered, the fraction of folded conformers diminishes, much like to what has been demonstrated by Laufen et al . [7] On the other hand, when the DnaJ/DnaK ratio increases to equimolar, the stabilization of unfolded conformers decreases and the fraction of misfolded conformers increases. This could explain why the intracellular concentration of DnaJ varies little even under heat-shock conditions [28] . Interestingly, under heat-shock conditions, the DnaJ/DnaK ratio decreases via further production of DnaK, which will in turn increases the fraction of arrested denatured substrates and provides an important protective role at the expense of folded conformers, while reducing aggregation to a minimum. We conclude that DnaK, although being modulated by DnaJ, has a crucial role in reducing misfolding under the crowded conditions of the cell. We further observed that GrpE slightly increases both the folded and misfolded populations while significantly decreasing the unfolded state ( Fig. 5 ). This finding is consistent with accelerated substrate release from DnaK [5] . Previous publications addressing the role of GrpE in the overall folding efficiency of the Hsp70 chaperone system render different results depending on the substrate used [29] , [30] . Thus, it may be considered that the optimal GrpE activity in the context of the Hsp70 chaperone system may be observed at different DnaJ/DnaK/GrpE ratios than that tested here. Here, our single-molecule refolding studies may offer a unique assay for fully addressing the GrpE functionality. The results presented are summarized in Fig. 6 . I27 domains can leave the unfolded state and reach folded or misfolded states through folding or misfolding pathways, respectively ( Fig. 6a ). DnaJ restricts the misfolding pathway by limiting the conformational space surrounding unfolded conformers ( Fig. 6b ). This directs unfolded substrates towards the productive folding pathway. Unlike with DnaJ alone, only when DnaK synergizes with DnaJ, misfolding can be fully suppressed ( Fig. 6c ). It is known that the presence of DnaJ and non-native substrate accelerates ATP hydrolysis by DnaK [7] , which triggers conformational changes that lead to non-covalent substrate entrapment by DnaK [31] . Therefore, we show that substrate entrapment by DnaK is accompanied by a stabilization of the unfolded state and an effective protection from aggregation. Because DnaJ together with DnaK efficiently suppresses misfolding, the unfolded substrate can thus only remain unfolded or travel along folding pathways. The trapped unfolded substrate, however, would require GrpE to be mobilized. 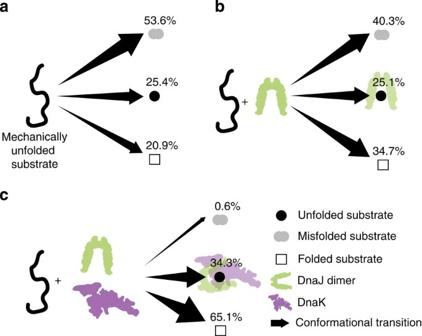Figure 6: Folding and misfolding pathways of unfolded I27 domains in the absence of chaperones, in the presence of DnaJ and in the presence of DnaJ and DnaK. (a) In the absence of chaperones, mechanically unfolded I27 domains (black curved line) can fold (white squares), remain unfolded (filled black circles), or aggregate and misfold (grey symbol). (b) In the presence of DnaJ, the conformational space of unfolded I27 is constrained. This constraint restricts the misfolding pathway and increases the probability for I27 domains to fold. (c) When DnaJ synergizes with DnaK in the presence of ATP, unfolded substrates are constrained and sequestered, thus stabilizing unfolded substrates to be processed. Accordingly, I27 can adopt the unfolded or the folded state, the latter representing the more stable conformer. Values presented were obtained from steady-state refolding experiments (tr=5 s) conducted in the absence of chaperones (a), the presence of 10 μM DnaJ (b) and in the presence of a 1:2 ratio of DnaJ/DnaK (5 μM DnaJ and 10 μM DnaK;c). The thickness of an arrow scales roughly to the probability of the conformational transition. Figure 6: Folding and misfolding pathways of unfolded I27 domains in the absence of chaperones, in the presence of DnaJ and in the presence of DnaJ and DnaK. ( a ) In the absence of chaperones, mechanically unfolded I27 domains (black curved line) can fold (white squares), remain unfolded (filled black circles), or aggregate and misfold (grey symbol). ( b ) In the presence of DnaJ, the conformational space of unfolded I27 is constrained. This constraint restricts the misfolding pathway and increases the probability for I27 domains to fold. ( c ) When DnaJ synergizes with DnaK in the presence of ATP, unfolded substrates are constrained and sequestered, thus stabilizing unfolded substrates to be processed. Accordingly, I27 can adopt the unfolded or the folded state, the latter representing the more stable conformer. Values presented were obtained from steady-state refolding experiments ( t r =5 s) conducted in the absence of chaperones ( a ), the presence of 10 μM DnaJ ( b ) and in the presence of a 1:2 ratio of DnaJ/DnaK (5 μM DnaJ and 10 μM DnaK; c ). The thickness of an arrow scales roughly to the probability of the conformational transition. Full size image Assessing the I27 sequence for DnaJ- and DnaK-binding sites Based on previously published work [14] , [32] , the amino-acid sequence of I27 was analysed for potential binding sites for DnaJ and DnaK using a custom-made algorithm built with ‘Igor 6.0’ (Wavemetrics). The algorithm first searches for hydrophobic core sequences consisting of four to five hydrophobic residues for DnaK-binding sites and four hydrophobic residues for DnaJ-binding sites. Thereafter, the vicinities of the hydrophobic core are equated and the algorithm searches for basic residues flanking up to four positions on each side of the hydrophobic core for DnaK-binding sites and searches for hydrophobic residues flanking up to two positions on each side of the hydrophobic core for DnaJ-binding sites. The relative frequencies in amino-acid content of chaperone-binding sites were provided by Rüdiger et al . for DnaK- [32] and DnaJ- [14] binding sites and used for computing a score reflecting the propensity for chaperones to bind to that specific amino-acid sequence. I27 sequences found for potential DnaJ-binding sites are: EKPLYGVE, KPLYGVEV, VEVFVGET, CQPLAASP, KHILILHN. The core sequence PLYGV renders the highest propensity for a DnaK-binding site. Preparation of gold supports Gold supports were prepared for tethering C-terminal cysteine residues of the 8xI27 construct as described [33] . Briefly, custom-made circular glass supports of 0.5 mm thickness and 4 mm radius (Huber & Co. AG) were glued to glass slides using epoxy resin (Epotek). The glued glass assembly was heated for 1–2 h at 120 °C and thereafter cleaned with 99% ethanol, distilled water and blow dried with N 2 . Gold was sputtered on sheets of mica by applying a 100-mA current for 180 s in vacuum after the sputter chamber was washed with argon. From sputtered mica sheets, segments were cut so that they were slightly larger than the circular glass supports. Thereafter, the gold-sputtered mica was glued to the circular glass supports, with the gold-coated side facing downwards, using epoxy resin (Epotek), and heated for 1–2 h at 120 °C. Before adsorbing the I27 sample to the gold support, mica was peeled off with tweezers and assessed for electrical conductivity with a multimetre. The electrodes were previously washed with 99% ethanol. Engineering of the I27 construct I27 sequence analysis were performed using DNA Strider [34] and ApE plasmid editor ( http://biologylabs.utah.edu/jorgensen/wayned/ape/ ). The expression plasmid pRSET A, containing 8xI27, was kindly provided by Jane Clarke [35] . Vector amplification of the expression plasmid was carried out in XL1-Blue competent cells (Strategene). Transformation was done through heat-shock treatment using 10 ng of the pRSET A vector. Plating was done on LB-ampicillin agar plates. The expression plasmids were transformed into E. coli BL21 strain. Cells were grown in lysogeny broth (LB) medium at 37 °C to an OD600 of 0.4–0.6 cm −1 . Expression was induced by addition of 0.2 mM isopropyl-β- D -thiogalactoside. Then, cells were grown overnight at 37 °C before harvesting by centrifugation. Cells were resuspended in phosphate-buffered saline (PBS), 10 mM sodium phosphate buffer, pH 7.4, 150 mM NaCl, and processed by high-pressure homogenizing (EmulsiFlex-C5, AVESTIN) on ice. Following centrifugation, the supernatant was incubated with a Ni-affinity matrix (Qiagen), which then was washed thoroughly with PBS (with 20 mM imidazole) followed by 50 mM Tris at pH 8.0. It then was eluted with 250 mM imidazole. A liquid chromatography purification step was added using a Sephadex G-200 column (Pharmacia) in an ÄKTA explorer 10S (Amersham Pharmacia) with PBS. Purification of DnaJ, DnaK and GrpE DnaJ was purified from overproducing strains of E. coli [10] . Briefly, cells were grown at 42 °C for 3 h in LB medium in the presence of 100 μg ml −1 ampicillin and 20 μg ml −1 chloramphenicol and harvested through centrifugation. The cell pellet was thereafter resuspended in 1 M KCl, 2 M urea and 0.1% Triton X-100, and subjected to a two-step purification protocol using DEAE-Sephacel and ammonium sulfate precipitation. To ensure more than 95% purity, chromatography was performed using first hydroxylapatite and then P-11-cellulose phosphate. DnaK was purified from ΔdnaK52 cells carrying a plasmid encoding wild-type DnaK [36] . Briefly, cells were grown at 37 °C and harvested through centrifugation. Thereafter, cells were resuspended in 180 mM spermidine-HCl., 50 mM dithiothreitol, 50 mM EDTA, 0.9 M ammonium sulfate and 2 mg ml −1 lysozyme. Protein precipitation was done by adding 280 g l −1 of ammonium sulfate followed by centrifugation. The resulting pellet was resuspended in 10 ml of a buffer containing 25 mM imidazole, pH 7.0, 10% sucrose, 25 mM NaCl, 5 mM MgCl 2 and 5 mM 2-mercaptoethanol, dialysed extensively, and applied to a 2 ml heparin/agarose column. The flow-through was then repeatedly applied to a 2.5-ml ATP/agarose column. The fraction containing the highest concentration of protein was applied to a Sephadex 75 column. Thereafter, the eluate was applied to a 1-ml Mono Q column. GrpE was purified from overproducing strains of E. coli [37] . Briefly, cells were grown in LB medium at 37 °C, harvested by centrifugation and thereafter lysed in a solution containing 46 pg ml −1 spermidine, 50 mM dithiothreitol, 50 mM EDTA, 1.5 M ammonium sulfate and 20 mg ml −1 lysozyme. The lysate was centrifuged two more times, with a decanting step in between. Thereafter, the supernatant was dialysed and applied to a DnaK affinity column. Protein concentrations were determined by quantitative amino-acid analysis. Sample preparation and cantilever calibration 8xI27 was diluted to a final concentration of 3.16 μM in a buffered solution consisting of 150 mM KCl, 5 mM MgCl 2 and 50 mM Tris-HCl pH 7.4 (refs 19 , 38 ). The protein solution was applied to a gold support, and incubated for 15 min at room temperature [39] . After adsorption to the support, 8xI27 was covalently tethered to the gold support through cysteine residues located at the C-terminus. This attachment leaves the N-terminus free to interact with the tip of the AFM cantilever [39] . Five washing steps followed with the same buffer to remove unbound protein. Refolding experiments were performed on the fully automated AFM ‘ForceRobot 300’ (JPK Instruments) [40] using a 3-port small volume ‘SmallCell’ (JPK), the 200-μm-long OMCL-RC800 cantilever (Olympus) showing a resonance frequency of 18 kHz in liquid, and a custom-made O-ring designed for long experimental times (maximum 36 h) while ensuring minimum evaporation. To increase their adhesiveness, cantilevers were bathed for 1 h in freshly prepared piranha solution (3:1 ratio of H 2 SO 4 /H 2 O 2 ). Cantilevers were calibrated using the thermal fluctuation method revealing an average spring constant ( k c ) of ≈55 pN nm −1 (refs 41 , 42 ). AFM protocol for automated refolding of 8xI27 To study the refolding of 8xI27 using AFM-based SMFS, we performed refolding experiments comprised by two unfolding segments performed at constant speed (1,200 nm s −1 ) and separated by a pause segment. In the first unfolding segment, a single 8xI27 was mechanically unfolded. After the first unfolding segment, 8xI27 was brought close to the support to remove the mechanically applied strain and to allow the unfolded polypeptide to refold for a certain refolding time ( t r ) during the pause segment. After t r , the second unfolding segment commences and the same 8xI27 polypeptide is once again unfolded to detect which I27 domains of the formerly unfolded 8xI27 refolded. Variation of t r reveals how fast refolding of individual I27 domains occurred (for example, refolding kinetics) [20] . Refolding times ( t r ) tested were 0, 1, 2, 5 and 8 s. Supplementary Fig. 6 details the experimental procedure into 11 sections. Proper identification of the force baseline is fundamental for identifying positive refolding force curves. Section 1 sets the zero force baseline and section 11 certifies whether the cantilever returned to a resting position ( Supplementary Fig. 6a,b ). For any given z-position away from the support ( Supplementary Fig. 6 , section 1 and i), the piezoelectric actuator was instructed to extend until the cantilever touched the support and deflected 1 nN ( Supplementary Fig. 6 , section 2 and ii). After a 1-s pause to increase the attachment probability of 8xI27 to the AFM tip ( Supplementary Fig. 6 , section 3), the actuator was retracted a distance that encompasses the length of 8xI27 to be unfolded plus the cantilever deflection ( Supplementary Fig. 6 , section 4). 8xI27 was kept in the unfolded state for 3 s to allow chaperone binding to unfolded I27 domains ( Supplementary Fig. 6 , section 5, iii). If an 8xI27 was picked by the AFM tip and held, a constant deflection above the baseline was recorded ( Supplementary Fig. 6 , section 5). This allowed us to identify if 8xI27 detached from the AFM tip ( Supplementary Fig. 6b,c , section 5). Thereafter, the actuator was extended bringing the AFM tip back to the support for a distance equalling the length of unfolded 8xI27 ( Supplementary Fig. 6 , section 6, iv). Henceforth, this travelled distance will be addressed as refolding length ( z r ). We inserted a pause segment during which 8xI27 was allowed to fold, varying t r between 0 and 8 s ( Supplementary Fig. 6 , section 7, v). Thereafter, 8xI27 was once again unfolded by retracting the actuator by the distance z r ( Supplementary Fig. 6 , section 8) and held ( Supplementary Fig. 6 , section 9, vi). The AFM protocol finishes with a final retraction of ≈1 μm, thus detaching 8xI27 from the support or AFM tip ( Supplementary Fig. 6 , section 10, vii), whose respective force peak is highlighted with an ‘*’ on Supplementary Fig. 6b . Refolding experiments Different refolding experiments were performed on 8xI27 following the general protocol for automated refolding. Each experimental condition was repeated at least five times, that is, a minimum of five 8xI27 samples was prepared per experimental condition. Between 4,000 and 8,000 force curves were acquired with each sample preparation, being ≈0.5% of them usable on average. To find out whether individual I27 domains misfolded or aggregated, refolding experiments were performed using a refolding length that comprises little over a single I27 domain ( z r ≈40 nm) and t r between 1 and 5 s. To study 8xI27 folding, experiments were performed with z r ≈185 nm, thus usually unfolding six to seven I27 domains in the first unfolding segment, although force-distance curves with five or even eight unfolded domains do occur. Nonetheless, the average number of I27 domains unfolded in the first unfolding segment is similar for all experimental conditions tested, thus dismissing possible concerns about its influence on the probability of refolding ( Supplementary Table 3 ). Refolding kinetics were investigated using t r between 1 and 8 s. The steady state of refolding of 8xI27 was found at t r of 5 s ( Supplementary Fig. 2 ). Single refolding experiments at steady state ( z r ≈185 nm , t r =5 s) were performed in the presence of members of E. coli Hsp70 system using 8xI27 as substrate. The conditions tested were: 1, 5, 10 and 20 μM DnaJ without ATP; 10 μM DnaK in the presence of ATP; 10 μM DnaJ and 0.1 μM DnaK in the presence of ATP; 10 μM DnaJ and 5 μM DnaK in the presence of ATP; 10 μM DnaJ and 10 μM DnaK in the presence of ATP; 10 μM DnaK, 10 μM DnaJ and 20 μM GrpE in the presence of ATP. Refolding experiments at steady state were performed in the presence of 20 μM lysozyme to account for the specificity of the experiments conducted with chaperones and to control for unspecific substrate–surface interactions as lysozyme readily adsorbs to gold [43] , [44] . The gold adsorption constant for lysozyme was calculated to be between 0.06 and 0.08 (ref. 44 ), implying that ≈100–125 ng of lysozyme are enough to cover the entire surface of the gold support (0.5 cm 2 ). This coverage of the surface leaves still enough protein in solution to control for chaperone activity (the effective concentration of lysozyme in solution would then be ≈18.5 μM). Analysis algorithms Channels corresponding to force ( F ), piezoelectric actuator’s displacement ( z ) and time ( t ) were exported for each force curve. An algorithm for automated sorting of force curves was applied using ‘Igor 6.0’ (Wavemetrics). Briefly, the algorithm searched for deviations from the force baseline in unfolding segments ( Supplementary Fig. 6 , sections 4 and 8), the presence of a constant deflection above the baseline during the section intended for chaperone binding ( Supplementary Fig. 6 , sections 5 and 9), the linear dropping in force upon re-approaching the support ( Supplementary Fig. 6 , section 6) and the positioning of the pause segment ( Supplementary Fig. 6 , section 7) relative to the force baseline ( Supplementary Fig. 6 , sections 1 and 11). An algorithm for semi-automatic data processing was also created in ‘Igor’. Briefly, sorted force curves are imported and the tip-sample separation ( x p ) channel is determined according to equation (1), where d is the cantilever deflection. Two force-distance curves are created corresponding to the first and second unfolding segments, that is, unfolding curve and refolding curve, respectively. Both force curves are first aligned with each other, and then aligned to a control 8xI27 force curve. Thereafter, an analysis routine is used to fit force peaks using the worm-like chain model described in equation (2), where k b is Boltzmann’s constant, T the absolute temperature, P the polymer’s persistence length and L the contour length [45] . Fits were performed with a P value of 0.4 nm. The output results are F , L , the difference in L between adjacent force peaks (Δ L ) and a string ‘ class ’ that classifies the adopted conformation. Three different conformations can be achieved by I27 domains ( Fig. 1c and Fig. 2a ): the I27 domain can refold into its native-like folded conformation; the I27 domain can form misfolded conformations; the I27 domains may not depart from the unfolded state. The folded conformation can be easily identified in 8xI27 as the protein exhibits a pattern of force peaks with a well-defined range of values for F and Δ L . Criteria were set based on force curves recorded from the first mechanical unfolding segment, where folded I27 domains present Δ L values between 25 and 31 nm ( Supplementary Fig. 1c ) and F values between 50 and 300 pN ( Supplementary Fig. 1d ). Force features that do not meet these criteria are considered the result of misfolding. The absence of force features for the remaining unfolded length means that the corresponding I27 domains did not refold and are therefore in the unfolded conformation ( Fig. 1b,c ). For each force-distance curve unfolded, misfolded and folded conformers are counted, and the resulting individual fractions are then averaged according to refolding time and experimental condition. Respective Δ L distributions for misfolded conformers are also determined. Statistical analysis After obtaining average fractions for folded, misfolded and unfolded conformers for each experimental condition, the distribution was subjected to the Shapiro–Wilk test to establish whether the data obtained came from normally distributed populations [46] . The results, summarized in Supplementary Table 1 , reveal that the great majority of data sets do not belong to a normal distribution. Furthermore, data sets were unsuccessfully subjected to a Box-Cox power transformation in an attempt to make it normally distributed. Therefore, a two-tailed Mann–Whitney U -test was performed to test the null hypothesis that two populations are the same [47] . P values are given in Supplementary Table 2 . How to cite this article: Nunes, J. M. et al . Action of the Hsp70 chaperone system observed with single proteins. Nat. Commun. 6:6307 doi: 10.1038/ncomms7307 (2015).